Homeostatic regulation of dendritic dynamics in a motor mapin vivo Neurons and circuits are remarkably dynamic. Their gross structure can change within minutes as neurons sprout and retract processes to form new synapses. Homeostatic processes acting to regulate neuronal activity contribute to these dynamics and predict that the dendritic dynamics within pools of neurons should vary systematically in accord with the activity levels of individual neurons in the pool during behaviour. Here we test this by taking advantage of a topographic map of recruitment of spinal motoneurons in zebrafish. In vivo imaging reveals that the dendritic filopodial dynamics of motoneurons map onto their recruitment pattern, with the most electrically active cells having the lowest dynamics. Genetic reduction of activity inverts this map of dynamics. We conclude that homeostatic mechanisms driven by a gradient of activity levels in a pool of neurons can drive an associated gradation in neuronal dendritic dynamics, potentially shaping connectivity within a functionally heterogenous pool of neurons. Neurons in the developing nervous system search for synaptic input by rapidly extending filopodia from their dendrites [1] , [2] , [3] , [4] , [5] , [6] , [7] , [8] , [9] , [10] , [11] , [12] , [13] . These filopodia are stabilized by molecular cues and activity from presynaptic axons, which in turn leads to synapse formation and subsequent dendritic growth [13] . In the absence of appropriate presynaptic partners the filopodia are retracted within a few minutes. Filopodial dynamics are high early in life, but decrease as neurons mature, presumably as a result of the increase in synaptic input [14] . Experimentally decreasing the amount of presynaptic input, or suppressing the activity of a neuron leads to larger dendritic arbours [15] , [16] . Conversely, increasing presynaptic input or making neurons more excitable leads to smaller dendritic arbours [15] , [16] , [17] . These observations lend support to the idea that dendritic arbours are homeostatic devices that grow in part to increase or decrease the synaptic input to neurons to achieve a particular level of activity. They lead to the prediction that if there were variations in the levels of activity in pools of neurons, there would be an associated variation in the dynamics of their dendrites that reflects their differing drive to find synaptic inputs. To explore this possibility, we took advantage of a recently discovered topographic map of recruitment and activity levels of spinal motoneurons in larval zebrafish [18] . Rapid time lapse imaging of dendritic arbours of neurons at different locations in the topographic map reveals that the dynamics vary systematically in a way that maps onto the recruitment and associated activity levels of these neurons. Older dorsal motoneurons, which are recruited rarely and only during the fastest movements, are more dynamic than younger, ventral motoneurons, which are recruited during movement at all speeds. We directly test a role for activity in setting up this pattern of dendritic dynamics by genetically reducing the excitability of individual neurons in an otherwise normal animal. Reducing excitability inverts the relationship between filopodial dynamics and location in the map as predicted by homeostatic considerations. Our work reveals that the dendritic dynamics of neurons in an intact nervous system map onto their activity level and behavioural role. This homeostatic matching of dynamics to function could ensure that the developmental phenomena that establish connectivity within a heterogeneous pool of neurons are appropriately tied to the functional roles of the individual neurons. Growth rates of motoneuron dendrites map to soma position Spinal motoneurons in zebrafish are systematically recruited from ventral to dorsal as the speed of swimming increases [18] , as illustrated in Fig. 1a . Once a motoneuron is recruited, it stays active at higher movement speeds, as in other vertebrates [19] , so the ventral neurons initially recruited at low speeds are active at all speeds, whereas dorsal ones are active just during the fastest movements. The result is an activity gradient, with the most active neurons located ventrally, and increasingly less active ones stacked in order above them. This orderly arrangement along with the transparency of zebrafish offers a powerful and unique opportunity to explore the relationship between variation in activity levels during normal behaviour and variation in dendritic dynamics in a pool of neurons whose behavioural roles are known. 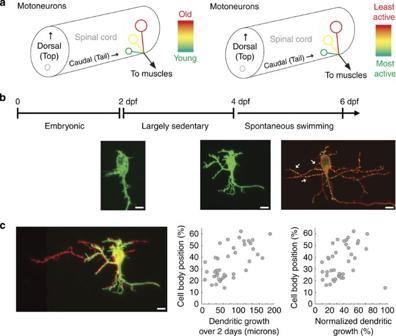Figure 1: Topographic organization of dendritic growth patterns. (a) Schematic summarizing the age-related dorsoventral organization of motoneurons in the spinal cord of zebrafish larvae. The youngest motoneurons are located in ventral spinal cord with older motoneurons occupying progressively more dorsal locations. This organization correlates with a gradient in the recruitment of motoneurons such that the youngest motoneurons are recruited most often, during movements of all speeds, whereas the older, more powerful dorsal motoneurons are recruited less frequently at only high speeds. (b) Images of motoneuron dendrites labelled with mGFP at 2 and 4 dpf. Right panel shows a motoneuron co-expressing PSD-95 (post synaptic density 95) tagged with GFP to mark glutamatergic synapses and a membrane-targeted Cherry (mMCherry) to highlight the dendritic arbour. Arrows point to filopodia-like structures without PSD-95 puncta. (c) Growth of motoneurons between 4 and 6 days. Left panel shows an overlay of the dendritic arbour of an individual motoneuron at 4 (green) and 6 days (red). Middle panel shows the relationship between the dendritic length added between 4 and 6 days and the dorsoventral position of the motoneuron. Right panel shows the dendritic growth between 4 and 6 days as a percentage of the total dendritic length at 4 days. Scale bar, 5 μm inb,c. Figure 1: Topographic organization of dendritic growth patterns. ( a ) Schematic summarizing the age-related dorsoventral organization of motoneurons in the spinal cord of zebrafish larvae. The youngest motoneurons are located in ventral spinal cord with older motoneurons occupying progressively more dorsal locations. This organization correlates with a gradient in the recruitment of motoneurons such that the youngest motoneurons are recruited most often, during movements of all speeds, whereas the older, more powerful dorsal motoneurons are recruited less frequently at only high speeds. ( b ) Images of motoneuron dendrites labelled with mGFP at 2 and 4 dpf. Right panel shows a motoneuron co-expressing PSD-95 (post synaptic density 95) tagged with GFP to mark glutamatergic synapses and a membrane-targeted Cherry (mMCherry) to highlight the dendritic arbour. Arrows point to filopodia-like structures without PSD-95 puncta. ( c ) Growth of motoneurons between 4 and 6 days. Left panel shows an overlay of the dendritic arbour of an individual motoneuron at 4 (green) and 6 days (red). Middle panel shows the relationship between the dendritic length added between 4 and 6 days and the dorsoventral position of the motoneuron. Right panel shows the dendritic growth between 4 and 6 days as a percentage of the total dendritic length at 4 days. Scale bar, 5 μm in b , c . Full size image The earliest born motoneurons in zebrafish, called primary motoneurons, differentiate at about 15–17 h post fertilization (hpf) and occupy the dorsal most position in the motor column [20] . Later born secondary motoneurons are added subsequently and are stacked below the primary motoneurones [21] . This age-related pattern of organization is also evident in spinal premotor interneurons that provide excitatory drive to motoneurons [22] . By 4 days post fertilization, the fish have hatched and are free swimming, with motoneurons recruited topographically with swimming speed from young ventral neurons to old dorsal ones as swimming frequency rises [18] . We explored the dendritic structure of these motoneurons by labelling individual cells by transient expression of membrane-targeted green fluorescent protein (GFP) driven by a Gal4 UAS system [23] with a bacterial artificial chromosome (BAC) for the zebrafish vesicular acetylcholine transporter (VAchT) driving Gal4, and UAS membrane-targeted GFP. This leads to a complete labelling of the neuron and allows for a three-dimensional (3D) examination of the entire dendritic arbour and its dynamics over time by using confocal imaging of the intact, living transparent fish. Initially, we examined when during development the dendrites were elaborated. 3D reconstructions from live fish showed that motoneurons at all dorsoventral locations in the motor column had not elaborated dendrites by 2 days post fertilization ( Fig. 1b ), but rather had only thin, dynamic filopodial processes, which are known to extend and retract as neurons search for synaptic inputs [4] , [11] , [13] . Fish hatch from the egg a day later at 3 days post fertilization and by 4 days they are swimming to find food and avoid becoming food, just as they must throughout the rest of their life. At 4 days, motoneurons throughout the dorsoventral extent of motor column have elaborated dendritic arbours. These arbours continue to grow indefinitely because fish, like most vertebrates, have indeterminate growth and so usually increase in size throughout life. We found that there is a topographic pattern to the growth in the motor pool, with the more active ventral motoneurons growing significantly less quickly than dorsal ones, even over a 2-day period in 4–6-day-old fish ( Fig. 1c ). One possible driver of the growth differences is homeostatic processes regulated by the levels of activity of a cell. Prior work revealed that an individual identifiable neuron in Drosophila compensates for perturbations of its synaptic input by increasing or decreasing its dendritic arbour [15] , [16] . When behaviour is instead driven by a pool of neurons, as is typically the case among vertebrates, natural variations in activity levels within the pool of neurons might drive processes that lead to synapse formation and dendritic growth and thus shape differences in connectivity in the pool. We therefore moved next to examine the unexplored question of how activity might shape dynamics and growth in a pool of neurons. Filopodial dynamics map on to motoneuron topography The growth of dendrites in zebrafish and xenopus tadpoles is accomplished by thin dynamic, filopodial extensions, which are constantly extending and retracting from the dendrites. Synaptic inputs onto a subset of the filopodia stabilize the process to form a new dendritic branch, which then serves as a source for new filopodial extensions to extend the arbour still further [11] , [13] , [24] . By labelling the motoneurons in zebrafish with both membrane-targeted mCherry and GFP-tagged PSD-95, we observed that the dendritic arbours of swimming age fish (4–6 days post fertilization (dpf)) had large and stable processes that contained PSD-95 puncta. Thinner, very dynamic filopodia arose from these dendrites, (see 1b, right). Repeated confocal imaging of the filopodia showed that most extended and then retracted within 5 min. A few, however, extended and remained extended for the duration of our imaging session (up to 30 min), consistent with evidence from other parts of the nervous system of zebrafish [13] and frog tadpoles [1] , [14] , [25] for a role of stabilized filopodia in dendritic growth. We explored the relationships between the positions of motoneurons, which reflect their age and activity level, and their dendritic structure and filopodial dynamics to test the hypothesis that dendritic dynamics were correlated with both activity levels and growth rate, with the prediction that more active ventral cells would be searching less vigorously for inputs, and, in turn, growing less. The dendritic arbours and filopodial dynamics of 34 motoneurons at different dorsoventral locations in 4 dpf fish were imaged every 5 min for 30 min ( Supplementary Movie S1 ). The filopodial lengths were measured in 3D for all neurons and time points, with tracking of individual filopodial extensions and retractions over the half hour period, as in the examples shown in Fig. 2a–h . A plot of the total stable (over the 30 min imaging period) length of the dendritic arbour of a motoneuron at 4 dpf against its dorsal ventral position in Fig. 2k showed that the ventral, youngest motoneurons tended to have the shortest total dendritic lengths. Dendritic length increased from ventral to dorsal in the motor map, with the most dorsal, oldest and least active neurons having the most extensive dendritic arbours ( n =34; P =0.0087). Both are not surprising because they are consistent with the overall faster growth of more dorsal, older and less active cells. Figure 2: Dendritic dynamics vary systematically with soma position in spinal cord. ( a , b ) Images of a ventral motoneuron expressing mGFP at the first two consecutive time points (0 and 5 min). ( c ) Overlaid image of a and b . Arrows point to filopodial extensions. ( d ) Reconstruction (in white) of dendritic extensions over a 30-min period in the same neuron. ( e , f ) Images of a dorsal motoneuron at the first two consecutive time points (0 and 5 min). ( g ) Overlaid image of e , f . Arrows point to filopodial extensions. ( h ) Reconstruction (in white) of the neuron’s filopodial extensions over a 30-min period. ( i , j ) Quantification of filopodial extensions and retractions between consecutive time points for 34 mGFP expressing motoneurons. Each row represents a single cell and the rows are arranged from bottom to top based on the ventral to dorsal position of the cell in the spinal cord. Each column represents the total length of filopodial extension between two consecutive time points normalized to the dendritic arbour length of that cell. Colour map is on the right. ( k ) Plot of cell body position versus length of dendritic arbour that remained unchanged over the entire imaging period for each motoneuron. Locations are normalized with respect to the dorsal (one) and ventral (zero) edges of spinal cord in all figures. ( l ) Plot of cell body position versus total number of filopodia extended in the 30-min imaging period. ( m ) Plot of position versus the summed length of all filopodial extensions over the entire imaging period. ( n ) Plot of soma position versus the normalized filopodial dynamics, which were calculated by dividing the sum of all filopodial extensions for a cell by the stable dendritic arbour length of that cell. Scale bar, 10 μm in a – h . Full size image The filopodial dynamics also mapped systematically onto motoneuron position and therefore the associated activity levels. Figure 2i show in a colour coded form the total length of the extensions or retractions in each 5 min interval for every motoneuron as a per cent of its total dendritic arbour length. The more dorsal neurons, in the upper rows, have higher dynamics, represented by the hotter colours in the diagram. A plot of the total number of filopodia extended over the 30 min period versus the dorsoventral location of a neuron, in Fig. 2l , shows that dorsal cells have systematically more total filopodial extensions than ventral ones ( n =34; P <0.0001). If the total length of extensions over the 30 min for each cell is plotted as a function of its dorsoventral location, as in Fig. 2m , there is also a significant correlation, with the dynamics increasing from ventral to dorsal ( n =34; P <0.0001). These relationships persist when the dynamics are normalized to the total dendritic arbour length of the neuron, Fig. 2n , to remove the possibility that bigger, more dorsal neurons have greater dynamics simply because they have more dendritic length from which extensions can arise ( n =34; P =0.0012). In summary, measures of both the total number of filopodial extensions in 30 min as well as the total length of new filopodia extended during that time showed that the ventral neurons were the least dynamic, with dendritic dynamics rising at increasingly more dorsal positions in spinal cord. Kir2.1 expression inverts the gradient of filopodial dynamics These observations raise the possibility that a gradient of activity levels in the pool drive a gradient of dendritic dynamics via homeostatic mechanisms and that these in turn contribute to a gradient of overall growth and the resulting variation in dendritic arbour sizes. If homeostatic mechanisms based upon activity levels do indeed drive the pattern of dendritic dynamics in this motor map, we would predict that if we altered neuronal excitability within the map, we would alter the topographic relationship between position and dendritic dynamics. We tested this prediction directly by transiently expressing an inwardly rectifying potassium channel (Kir2.1) (ref. 26) [26] to sparsely label motoneurons, thereby lowering excitability in isolated motoneurons at different locations in the map in otherwise normal fish. The channel construct we used lowers the input resistance of neurons and reduces the activity level of zebrafish spinal neurons, as demonstrated by previous calcium imaging of Kir2.1 expressing spinal neurons in zebrafish [27] . We measured the dendritic filopodial dynamics and overall growth of the Kir2.1 expressing neurons, as we did the unperturbed cells. A non-conducting version of Kir2.1 with a mutated pore [26] was used as a control to tie any effects to the change in conductance rather than the effects of expressing this exogenous membrane protein. Expression of Kir2.1 dramatically altered the filopodial dynamics of neurons in the map in a manner predicted by homeostatic considerations ( Figs 3 , 4 ). The usually less dynamic, younger ventral motoneurons increased their dynamics substantially after Kir2.1 expression, as evident in individual neurons ( Fig. 3a–h ; Supplementary Movie S2 ), and in the heat maps of the summed lengths of extensions or retractions for all time points and all neurons ( Fig. 3i–j ). After the perturbation with Kir2.1, the normal increase in the number of extensions from ventral to more dorsal motoneurons, shown by the positive slope of the relationship in the grey dots on Fig. 4a , was altered significantly because of an increase in dynamics of the ventral neurons (red dots on 4a). The relationship between the total length of extensions and the location of a motoneuron also changed after Kir expression in a way consistent with a large increase in the dynamics of ventral neurons ( Fig. 4b ). Normalization of the summed filopodial extension lengths to the stable dendritic arbour length in individual motoneurons ( Fig. 4c ) revealed that Kir2.1 actually inverted the normal relationship between position and dendritic dynamics ( n =16; P =0.0017). The changes were also evident in the extent of retractions ( Fig. 4e–g ). After Kir2.1 expression, the level of both extensions and retractions decreased from ventral to dorsal rather than increasing. Neurons expressing non-conducting versions of the Kir2.1 channel showed dynamics that matched neurons expressing only membrane-tagged GFP (mGFP), indicating that a functional channel drove these changes in dendritic dynamics. Although the dynamics were dramatically affected by the perturbation, in contrast to work in other systems [15] , [16] , the neurons expressing the channel did not show a change in their total stable dendritic length at 4 days relative to motoneurons expressing just a membrane tag, or to ones expressing a non-conducting channel ( Fig. 4d ). Figure 3: Kir2.1 expression increases dendritic dynamics in ventral motoneurons. ( a , b ) Images of a ventral motoneuron expressing Kir2.1-viral2a-mGFP at the first two consecutive time points (0 and 5 min). ( c ) Overlaid image of a and b . Arrows point to filopodial extensions. ( d ) Reconstruction (in white) of dendritic extensions over a 30-min period. ( e , f ) Images of a dorsal motoneuron at the first two consecutive time points (0 and 5 min). ( g ) Overlaid image of e , f . Arrows point to filopodial extensions. ( h ) Reconstruction (in white) of filopodial extensions over a 30-min period. ( i , j ) Quantification of filopodial extensions and retractions between consecutive time points for 16 Kir2.1-viral2a-mGFP expressing motoneurons. Each row represents a single cell and the rows are stacked from bottom to top based on the ventral to dorsal position of the cell in the spinal cord. Each column represents the total length of filopodial extensions between two consecutive time points normalized to the dendritic arbor length of that cell. Colour map is on the right. Scale bar, 10 μm in a – h . 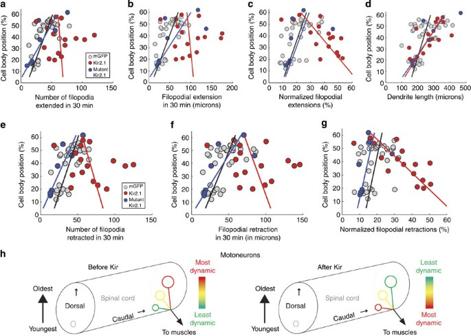Figure 4: Changing the excitability of motoneurons reverses the gradient of dendritic dynamics but does not affect stable dendritic size. (a) Plot of cell body position versus total number of filopodia extended in the 30-min imaging period for: 16 motoneurons expressing Kir2.1-viral2a-mGFP (red circles); 34 mGFP expressing motoneurons (grey circles); and 7 mutantKir2.1-viral2a-mGFP expressing motoneurons (blue circles). (b) Plot of position versus the sum of all filopodial extensions over the entire imaging period. (c) Plot of position versus filopodial dynamics normalized to the stable dendritic arbour length of the cell. (d) Plot of cell body position versus stable dendritic arbour length for each group. (e–g) Plots of retractions similar to those for extensions ina–c. (h) Schematic showing the inverted gradient of motoneuron dendritic dynamics as a consequence of decreasing the excitability of motoneurons. Full size image Figure 4: Changing the excitability of motoneurons reverses the gradient of dendritic dynamics but does not affect stable dendritic size. ( a ) Plot of cell body position versus total number of filopodia extended in the 30-min imaging period for: 16 motoneurons expressing Kir2.1-viral2a-mGFP (red circles); 34 mGFP expressing motoneurons (grey circles); and 7 mutantKir2.1-viral2a-mGFP expressing motoneurons (blue circles). ( b ) Plot of position versus the sum of all filopodial extensions over the entire imaging period. ( c ) Plot of position versus filopodial dynamics normalized to the stable dendritic arbour length of the cell. ( d ) Plot of cell body position versus stable dendritic arbour length for each group. ( e – g ) Plots of retractions similar to those for extensions in a – c . ( h ) Schematic showing the inverted gradient of motoneuron dendritic dynamics as a consequence of decreasing the excitability of motoneurons. Full size image Although the mechanistic aspects of dendritic dynamics have been well-studied [2] , [3] , [4] , [13] , [25] , [28] , we set out to fill an important gap in our understanding of how those dynamics relate to functional differences among neurons. Our work reveals a topographic pattern of dendritic dynamics within a pool of neurons that maps onto their orderly patterns of recruitment during behaviour. Motoneurons are recruited from ventral to dorsal with increases in swimming speed [18] , resulting in an activity gradient from high levels in very active ventral neurons to low levels in the rarely recruited dorsal ones. The dynamics map in a direction opposite to the activity map, with the lowest dynamics in the most active, ventral cells and the highest in the dorsal ones. If the dynamics are driven by activity, homeostatic considerations [26] , [29] predict that reducing the activity of ventral motoneurons would increase filopodial dynamics as they searched for inputs to restore their normally higher activity levels. This is what we found. The ventral neurons, with the highest activity levels and the lowest dendritic dynamics before the Kir2.1 expression, were most perturbed by lowering their excitability ( Fig. 4h ). Our evidence supports the conclusion that the normal topographic map of dendritic dynamics is driven at least in part by the topography of recruitment and the associated gradient of activity levels. Importantly, more active neurons in the pool are the least dynamic, even though they are the younger members of the pool, and might be expected to be growing the most if growth rate was based on age alone. The absence of a change in the overall stable dendritic size of the motoneurons after the perturbation indicates that increased filopodial dynamics are not sufficient for increasing total dendritic arbour size, even in the ventral neurons, which showed a large increase in filopodial dynamics after Kir expression. One possible alternative interpretation is that there was not sufficient time for the filopodial extensions to drive additional growth by 4 days of age, when we measured the arbour size. This is unlikely because the dendrites grow from almost nothing to substantial arbours between 2 and 4 days, so there is a major dendritic elaboration in this time period. This, combined with our data showing that the dorsal neurons elaborate substantially larger arbours than the ventral ones by 4 days, indicates that there is time for the increased filopodial dynamics to lead to elaboration of a larger arbour by 4 days of age. Apparently, the neurons searched more for inputs, but failed to find more than they did when searching at the normal, lower, unperturbed rate. An increase in dendritic arbour length likely requires exploratory activity of both pre [12] , [30] , [31] and post synaptic partners, appropriate molecular cues [32] , [33] , and stabilization of synapses by appropriate timing of neuronal activity [25] . As our perturbations exclusively manipulated single postsynaptic neurons in an otherwise normal population of cells, evidently all of the conditions for increasing dendritic arbour growth were not present. Instead, we revealed how neuronal activity influences dendritic dynamics in a cell autonomous fashion. The ability of activity to alter dynamics without affecting growth suggests that it may be important that the normal homeostatic drive of dendritic dynamics somehow be matched to the availability of inputs, so that the neurons are not searching more than necessary to achieve the appropriate rate of dendritic growth. Selective regulation of dynamics based on a neuron’s excitability and associated postsynaptic activity levels could be a simple but effective mechanism for ensuring that energetically expensive exploratory activity is restricted only to those neurons in a pool that need inputs the most. Taken together, our results show that a topographic map of activity in a pool of motoneurons is correlated with a corresponding topography of dendritic dynamics within the pool. Surprisingly, older neurons are more dynamic than younger ones, leading to the hypothesis that it is activity that drives the dynamics, not youthfulness, because older neurons are less active than young ones. Perturbations of excitability inverted the topography of dynamics in a way consistent with a role for a homeostatic, activity driven mechanism in setting up the patterns of dendritic dynamics in the motor pool. These cell autonomous, activity-dependent differences in the dendritic dynamics within a pool of neurons may act in conjunction with the availability of presynaptic inputs to optimally establish the appropriate patterns of dendritic growth and connectivity required for normal patterns of recruitment during behavior. Transient expression of a fluorescent reporter in motoneurons All procedures conform to the National Institutes of Health guidelines regarding animal experimentation and were approved by Cornell University’s Institutional Animal Care and Use committees. DNA was injected at low concentrations (20–30 ng μl −1 ), as previously described [34] , into fertilized eggs at the single-cell stage resulting in stochastic expression of fluorescent protein in isolated motoneurons. Embryos were screened for expression of fluorescence at 72–80 hpf and embryos with unambiguous individually labelled motoneurons were selected for imaging. In order to increase reporter expression levels, the Gal4-VP16/14XUAS system was utilized [23] . A BAC containing regulatory elements for the VAchT was modified by homologous recombination to create a VAchT:Gal4 driver to target expression to motoneurons. To drive the expression of membrane-targeted GFP, a 14X UAS :mGFP reporter construct was coinjected with VAchT:Gal4. The 14X UAS :mGFP construct was derived from 14XUAS [23] and brn3c:mGFP [35] . To drive the expression of Kir2.1 and membrane-targeted GFP in the same neuron, we used the viral2a [36] approach to co-express the two proteins. A 14X UAS Kir2.1-viral2a-mGFP construct was created using the Tol2 cloning approach [37] . A non-conducting version of Kir2.1, mut.Kir2.1, was constructed similarly to make the 14X UAS mutKir2.1-viral2a-mGFP construct. Details of the cloning are available on request. In vivo confocal microscopy Larvae were anaesthetized in a 0.02% solution of MS-222 and then paralysed by immersion in 1 mg ml −1 α-bungarotoxin (Sigma Co.) in 10% Hank’s solution without anaesthetic. Once larvae were immobilized (2–3 min), they were embedded in low melting-point agarose, covered in 10% Hank’s solution without anaesthetic, so that anaesthetic effects did not interfere with dendritic dynamics. Fish were oriented such that motoneurons were imaged from the lateral view. Hank’s solution was maintained at 28.5 °C for the duration of imaging. Labelled cells were imaged using an inverted confocal microscope (Zeiss LSM 510, Carl Zeiss) with a Zeiss C-Apochromat × 40 water lens. Green fluorescence was excited using 488 nm laser light and emission was typically collected with band pass emission filters (505–530 or 505–550 nm). For dendritic dynamics experiments, the entire dendritic arbour was imaged in 3D every 5 min for 30 min total. A subsequent image was collected where the dendritic structure was imaged simultaneously with a DIC image of the spinal cord to determine the dorsoventral location of the neuron in the spinal cord. Image processing and quantification 3D image rendering and analyses of dendrite dynamics were performed using Imaris (Bitplane, Inc.). Any drift during imaging was corrected by using the SPM Matlab toolbox and custom Matlab scripts that aligned the 3D z-stacks at each time point using the z-stack at the first time point as the reference. Some z-stacks were manually adjusted using the ‘Channel Shift’ function in Imaris to ensure that the images were well aligned. All aligned z-stacks were then smoothed by median filtering to aid in dendritic reconstruction. The images were checked manually to ensure that no obvious artifacts were introduced due to smoothing. For reconstructing filopodial extensions and retractions, 3D renderings of z-stacks from two consecutive time points were overlaid and pseudocolored red and green. Non-overlapping parts of the dendritic structure were drawn in 3D in Imaris (Filament function) and classified as extensions or retractions between the two time points. This was then done for every time point to quantify all of the extensions and retractions between consecutive time points. Blind analysis of coded data sets confirmed that the relationships we found were independent of any subjective bias in the analysis process. The reconstructed (stable) dendritic arbour was the dendritic arbour that was conserved over the entire imaging period. To obtain this, the dendritic arbour was reconstructed in 3D in Imaris (Filament function) using the first z-stack from the first time point as the reference. This reconstruction was then overlaid on a 3D rendering of the z-stack from the last time point and edited so that it represented the dendritic arbour that was conserved between the first and the last time point. Quantification of dorsoventral soma position The DIC image of the spinal cord was used to identify its ventral and dorsal edges. Motoneuron location was determined by averaging three measurements from the bottom of spinal cord to the middle of the cell body using Zeiss LSM 510 software. This value was then divided by an average of three measurements of the total dorsoventral extent of spinal cord to normalize the measurements, with the bottom of spinal cord equal to zero and the top equal to one. Statistics Correlations and the significance of the correlations were tested in Matlab with the corrcoef function. Comparisons of the effects of expression of Kir and mutant Kir with wild-type were done by using an analysis of covariance in JMP (SAS Institute). A level of 0.05 was used as the basis for significance. How to cite this article: Kishore S. et al. Homeostatic regulation of dendritic dynamics in a motor map in vivo . Nat. Commun. 4:2086 doi: 10.1038/ncomms3086 (2013).